Re-evaluating the phylogenetic position of the enigmatic early Cambrian deuterostomeYanjiahella 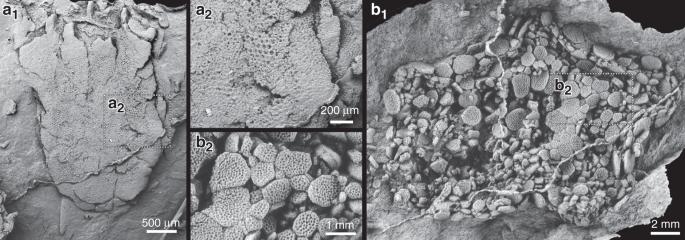Fig. 1: Latex casts of Cambrian echinoderms from the Jbel Wawrmast Formation (Morocco) showing relic “ghost” stereom microstructure associated with the presence of originally calcitic plates. aSEM image of a ctenocystoid with a loosely calcified ventral surface. Specimen NHMUK EE15317 (a1). General view (a2). Detail showing stereom in the surface of the plates.bVentral surface of an edrioasteroid. Photograph of latex cast whitened with ammonium chloride sublimate. Specimen NHMUK EE15308 (b1). General view.(b2). Detail of plate sutures and ornamentation. Specimens housed in the Natural History Museum, London (NHMUK). 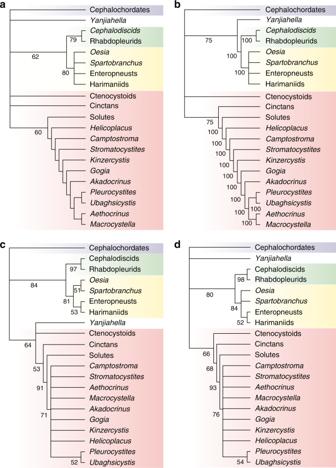Fig. 2: Phylogenetic uncertainty in placement ofYanjiahella. aStrict consensus of twelve most parsimonious trees (MPTs) recovered via maximum parsimony analysis of the matrix in Topper et al.3(including parsimony uninformative characters: tree length = 70, CI = 0.657; excluding parsimony uninformative characters: tree length = 63, CI = 0.619), node values = bootstrap support via 1,000 replicates.bparsimony-based 50% majority rule tree, node values = clade frequencies across MPTs.cBayesian 50% majority rule tree of the matrix in Topper et al.3, node values = posterior probability (%).dBayesian 50% majority rule tree from a matrix in whichYanjiahellais re-scored as lacking stereom (character 16), node values = posterior probability (%). Character matrices To quantify support for the phylogenetic placement of Yanjiahella , we re-analyzed the original matrix in the Supplemental Information of Topper et al. [3] using both maximum parsimony and Bayesian approaches. In contrast to Topper et al. [3] (cf. fig. 3 and Supplementary figs. 6 , 7 ), we present results matching each method’s respective optimality criteria (e.g., minimum-length trees for parsimony analysis) only. We also conducted analyses with Yanjiahella re-scored as lacking stereom (i.e., changing character 16 from “?” to “0”). We note that 7 of the 42 characters (~17%) used by Topper et al. [3] are not parsimony informative. Phylogenetic analyses Parsimony analyses were conducted in PAUP* 4.0a [12] using a heuristic search of 1,000 random addition sequence replicates with branch swapping via tree-bisection-reconnection. Branches with a minimum length of zero were collapsed. All characters were unordered and equally weighted. Bootstrap support was evaluated across 10,000 replicate matrices of the 35 parsimony-informative characters included in Topper et al. [3] . Summary statistics for the set of most parsimonious trees (MPTs) were calculated in PAUP* for both the total set of 42 characters and 35 parsimony-informative characters. To further compare our results with Topper et al.’s [3] figure 3, we also conducted analyses in TNT [13] using implicit enumeration with branch collapse settings off. Bayesian analyses were conducted in MrBayes 3.2.5 [14] using Markov chain Monte-Carlo (MCMC). We used the standard Mk model of morphological evolution with gamma distributed rate variation and a compound Dirichlet prior on branch lengths. Two runs of four MCMC chains were sampled every 5000 generations across 5 million generations, discarding the first 25% as burn-in. MCMC convergence was assessed using standard MrBayes diagnostics, including the standard deviation of clade frequencies and potential scale reduction factor [14] . Clade support was evaluated using posterior probabilities for nodes retained in the 50% majority rule consensus tree. Ancestral state reconstructions were conducted in Mesquite [15] . A batch file containing the data and scripts to reproduce our phylogenetic results is provided in Supplementary Data 1 . Reporting summary Further information on research design is available in the Nature Research Reporting Summary linked to this article.